Mondo complexes regulate TFEB via TOR inhibition to promote longevity in response to gonadal signals Germline removal provokes longevity in several species and shifts resources towards survival and repair. Several Caenorhabditis elegans transcription factors regulate longevity arising from germline removal; yet, how they work together is unknown. Here we identify a Myc-like HLH transcription factor network comprised of Mondo/Max-like complex (MML-1/MXL-2) to be required for longevity induced by germline removal, as well as by reduced TOR, insulin/IGF signalling and mitochondrial function. Germline removal increases MML-1 nuclear accumulation and activity. Surprisingly, MML-1 regulates nuclear localization and activity of HLH-30/TFEB, a convergent regulator of autophagy, lysosome biogenesis and longevity, by downregulating TOR signalling via LARS-1/leucyl-transfer RNA synthase. HLH-30 also upregulates MML-1 upon germline removal. Mammalian MondoA/B and TFEB show similar mutual regulation. MML-1/MXL-2 and HLH-30 transcriptomes show both shared and preferential outputs including MDL-1/MAD-like HLH factor required for longevity. These studies reveal how an extensive interdependent HLH transcription factor network distributes responsibility and mutually enforces states geared towards reproduction or survival. Pioneering work in model genetic organisms has led to the discovery of conserved signalling pathways that regulate animal longevity [1] . These pathways include reduced insulin/insulin growth factor (IGF) signalling, dietary restriction, reduced mitochondrial respiration, decreased target of rapamycin (TOR) signalling and signals from the reproductive system, which promote health and longevity through enhanced protein quality control, stress resistance, metabolic homeostasis and immunity. Molecular genetic experiments performed in C. elegans reveal that these pathways work through specific constellations of transcription factors. For example, the long life of reduced insulin/IGF signalling daf-2 /InsulinR mutants depends largely on the DAF-16/FOXO, SKN-1/NFE-2 and HSF-1 transcription factors [2] , [3] , [4] , whereas dietary restriction-induced longevity is mediated by PHA-4/FOXA, NHR-62/HNF4, SKN-1/NFE-2 and NHR-8/LXR [5] , [6] , [7] , [8] . Of particular interest is the gonadal longevity pathway. Removal of germline precursors results in a prodigious 60% increase in lifespan [9] , which depends on bile acid-like steroids emanating from the somatic gonad [10] , [11] , [12] . Virtually, every known longevity factor including the steroid receptor DAF-12/FXR, DAF-16/FOXO, HSF-1, NHR-80/HNF4, PHA-4/FOXA and NHR-49/PPARα function in this pathway [4] , [9] , [13] , [14] , [15] but how these factors cooperate in transcriptional networks is poorly understood. Dissecting such circuitry may reveal how regulatory functions are distributed and converge at key nodes within networks to establish signalling states and help pinpoint processes critical for longevity. Although the major longevity pathways behave independently by genetic criteria, a number of convergent processes have emerged in common. This includes the process of autophagy, the intracellular engulfment of protein aggregates, defective organelles and internal membranes, with delivery to the lysosome for turnover. Autophagy is necessary for longevity in many pathways and, in some cases, enhanced autophagy is sufficient to extend life [16] , [17] , [18] , [19] , [20] . HLH-30/TFEB transcription factor, recently shown to promote autophagy and lysosomal biogenesis [21] , [22] , also works in various longevity pathways, revealing a key regulator of core longevity mechanisms [19] . However, the regulatory cascades that govern these core longevity mechanisms remain unexplored. To uncover new regulators of the gonadal longevity pathway, we performed systematic RNA interference (RNAi) screens and discovered a key role for Myc superfamily members MML-1 (Myc/Mondo-like) and its partner MXL-2 (Max, Max-like) in mediating gonadal longevity, as well as longevity in other conserved pathways. Our studies suggest that MML-1 and MXL-2 work in transcriptional cascades that reduce TOR activity, which in turn stimulates autophagy and HLH-30/TFEB activity in the nucleus. Together, MML-1/MXL-2 and HLH-30 cooperate to extend life but also regulate distinct gene sets important for longevity. These studies illuminate a core regulatory network broadly affecting animal lifespan. mml-1/mxl-2 are required for multiple longevity pathways To identify new mediators of gonadal longevity, we performed RNAi screens encompassing ca . 600 transcription factors for suppressors of longevity in germline-less glp-1 mutants ( Fig. 1a ). We obtained previously known regulators such as daf-16 , daf-12 and hlh-30 , as well as several novel regulators including mml-1 and mxl-2 as potent candidates. MML-1 and MXL-2 belong to the Myc super family of basic helix-loop-helix (bHLH-Zip) E-box factors: MML-1 (Myc and Mondo-like) is homologous to MondoA/ChREBP, whereas MXL-2 is homologous to Max-like and works together with MML-1 in an activation complex [23] ( Fig. 1b ). In mammals, MondoA/Max-like and ChREBP (MondoB)/Max-like complexes respond to glucose and regulate glycolysis and lipogenesis [24] , [25] . 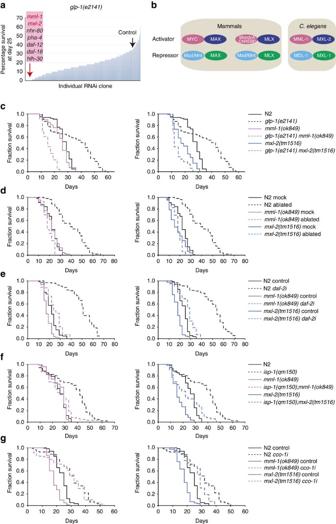Figure 1: MML-1/MXL-2 are required for multiple longevity pathways. (a)glp-1(e2141)suppressor screens identifymml-1andmxl-2as new transcription factors required for gonadal longevity. Survivorship ofglp-1(e2141)worms on control RNAi (L4440, black arrow) and experimental RNAi was determined at day 25. Knockdown of known factors (for example,daf-16,daf-12andhlh-30), as well asmml-1andmxl-2, completely suppressedglp-1survivorship. Survivorship of 60 worms was determined and screening conducted twice. (b)C. elegansMyc superfamily comprises MML-1/MXL-2 and MDL-1/MXL-1 complexes. (c–g) Roles ofmml-1andmxl-2in various longevity pathways.mml-1(ok849)andmxl-2(tm1516)deletions suppress longevity of germline-deficientglp-1(e2141)mutants (c) and animals with germline laser microsurgery (d).mml-1andmxl-2suppress longevity ofdaf-2RNAi (e).mml-1is required forisp-1 (qm150)longevity(f)but not required for the longevity conferred bycco-1RNAi (g).mxl-2is not specifically required forisp-1orcco-1RNAi longevity (f,g). SeeSupplementary Table 1for details and repeats. Figure 1: MML-1/MXL-2 are required for multiple longevity pathways. ( a ) glp-1(e2141) suppressor screens identify mml-1 and mxl-2 as new transcription factors required for gonadal longevity. Survivorship of glp-1(e2141) worms on control RNAi (L4440, black arrow) and experimental RNAi was determined at day 25. Knockdown of known factors (for example, daf-16 , daf-12 and hlh-30 ), as well as mml-1 and mxl-2 , completely suppressed glp-1 survivorship. Survivorship of 60 worms was determined and screening conducted twice. ( b ) C. elegans Myc superfamily comprises MML-1/MXL-2 and MDL-1/MXL-1 complexes. ( c–g ) Roles of mml-1 and mxl-2 in various longevity pathways. mml-1(ok849) and mxl-2(tm1516) deletions suppress longevity of germline-deficient glp-1(e2141) mutants ( c ) and animals with germline laser microsurgery ( d ). mml-1 and mxl-2 suppress longevity of daf-2 RNAi ( e ). mml-1 is required for isp-1 (qm150) longevity (f) but not required for the longevity conferred by cco-1 RNAi ( g ). mxl-2 is not specifically required for isp-1 or cco-1 RNAi longevity ( f , g ). See Supplementary Table 1 for details and repeats. Full size image Demographic analysis confirmed that mml-1 and mxl-2 deletions abolished lifespan extension in glp-1 mutants and in animals whose germline precursors were removed by laser microsurgery, while only modestly shortening wild-type lifespan ( Fig. 1c,d ). We also examined interactions with other longevity pathways and found that mml-1 and mxl-2 were largely required for daf-2 /InsR longevity ( Fig. 1e ), similar to previous reports [26] . In addition, mml-1 was partially required for isp-1 longevity but had little effect on longevity on cco-1 RNAi, whereas mxl-2 had little specific effect on either ( Fig. 1f,g ). Consistent with a role in longevity regulation, mml-1 overexpression in wild type sufficed to extend lifespan in three of six experiments ( Supplementary Fig. 1a and Supplementary Table 1 ) but did not further extend glp-1 longevity ( Supplementary Fig. 1b ). These findings indicate that mml-1 and mxl-2 work within several longevity pathways and have overlapping but distinct functions. Signals from the reproductive system regulate mml-1 A rescuing MML-1::GFP translational reporter ( Supplementary Fig. 1c ) was widely expressed and found in the cytoplasm and nuclei of the intestine, neurons, muscle, hypodermis, excretory cell and other tissues ( Supplementary Fig. 2a ) [23] . A closer examination of the subcellular localization revealed that MML-1::GFP also co-localized with the mitochondria, comparable to mammalian MondoA ( Fig. 2a ) [27] . A rescuing MXL-2::GFP translational reporter construct was also widely expressed and overlapped with MML-1 in most tissues ( Fig.2a and Supplementary Figs 1d and 2b ), but was distributed smoothly in the cytoplasm and nucleus, with only sporadic mitochondrial localization. Interestingly, we noticed that both mml-1 messenger RNA levels and MML-1::GFP nuclear accumulation were increased in glp-1 mutants ( Fig. 2b-d ). In contrast, MXL-2::GFP did not change on germline removal, although mxl-2 transcripts were increased ca . 1.5-fold ( Supplementary Fig. 2c–e ). Thus, mml-1 is visibly regulated in response to germline signalling. 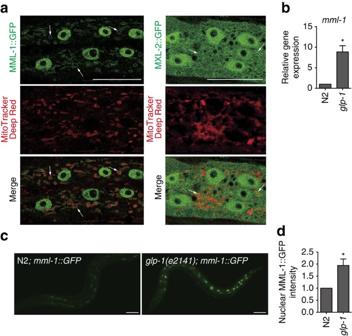Figure 2: MML-1 is regulated on germline removal. (a) MML-1::GFP and MXL-2::GFP (green) in hypodermal cells (wild type, L4 stage). MML-1::GFP is localized to the nucleus and the mitochondria (white arrows). MXL-2::GFP is not specifically localized, but occasionally overlapped with the mitochondria (white arrows). Mitochondria are marked by MitoTracker Deep Red (Red). (b)mml-1transcripts are upregulated inglp-1(e2141)animals relative to wild-type N2 as measured by qRT–PCR using total RNA samples prepared from >200 young adult worms. Mean±s.e.m. from three independent experiments are depicted and are normalized to wild-type N2.P-value (*P<0.05) was determined byt-test. (c) The representative fluorescent images ofmml-1::GFP transgenic worms in wild-type N2 andglp-1worms at day 1 young adult stage. Nuclear MML-1::GFP is elevated inglp-1animals. (d) Quantification of nuclear MML-1::GFP in the posterior intestinal nucleus at day 1 young adult stage. Mean±s.e.m. from four biological replicates (>20 worms each) relative to N2 are presented.P-value (*P<0.05) was determined byt-test. Two other independent MML-1::GFP transgenic lines show a similar tendency (not shown). Scale bars, 20 μm (a) and 50 μm (c). Figure 2: MML-1 is regulated on germline removal. ( a ) MML-1::GFP and MXL-2::GFP (green) in hypodermal cells (wild type, L4 stage). MML-1::GFP is localized to the nucleus and the mitochondria (white arrows). MXL-2::GFP is not specifically localized, but occasionally overlapped with the mitochondria (white arrows). Mitochondria are marked by MitoTracker Deep Red (Red). ( b ) mml-1 transcripts are upregulated in glp-1(e2141) animals relative to wild-type N2 as measured by qRT–PCR using total RNA samples prepared from >200 young adult worms. Mean±s.e.m. from three independent experiments are depicted and are normalized to wild-type N2. P -value (* P <0.05) was determined by t -test. ( c ) The representative fluorescent images of mml-1 ::GFP transgenic worms in wild-type N2 and glp-1 worms at day 1 young adult stage. Nuclear MML-1::GFP is elevated in glp-1 animals. ( d ) Quantification of nuclear MML-1::GFP in the posterior intestinal nucleus at day 1 young adult stage. Mean±s.e.m. from four biological replicates (>20 worms each) relative to N2 are presented. P -value (* P <0.05) was determined by t -test. Two other independent MML-1::GFP transgenic lines show a similar tendency (not shown). Scale bars, 20 μm ( a ) and 50 μm ( c ). Full size image Mutual regulation of MML-1 and HLH-30 The bHLH transcription factor HLH-30/TFEB is a conserved regulator of autophagy and lysosome biogenesis in C. elegans and mammals [19] , [21] , [22] . Similar to mml-1 , it is also required for multiple forms of longevity including gonadal longevity ( Supplementary Table 1 ). Notably, HLH-30/TFEB becomes nuclear localized in response to germline removal [19] . Given their phenotypic congruence, we asked whether there is a functional relationship between MML-1/MXL-2 and HLH-30. We found that deletion of mml-1 or mxl-2 dramatically impaired HLH-30::GFP nuclear accumulation in germline-less animals ( Fig. 3a,b and Supplementary Fig.3a ). Whereas >90% of glp-1 animals showed HLH-30::GFP nuclear localization, <15% of glp-1mml-1 and glp-1mxl-2 animals evoked this phenotype. Knockdown of mml-1 and mxl-2 also reduced HLH-30::GFP nuclear localization in daf-2 and eat-2 backgrounds ( Supplementary Fig. 3b,c ). By contrast, mml-1/mxl-2 had little effect on the expression of pha-4/ FOXA ( Supplementary Fig. 3d ) or nuclear localization of daf-16/ FOXO ( Supplementary Fig. 3e,f ), other important regulators of gonadal longevity. Moreover, hlh-30 RNAi knockdown significantly reduced the expression levels of MML-1::GFP in germline-less animals ( Fig. 3c,d and Supplementary Fig. 3g ). Therefore, MML-1 and HLH-30 mutually regulate one another. 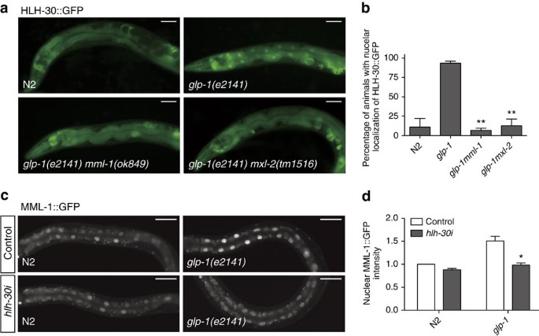Figure 3: Mutual regulation of MML-1 and HLH-30. (a) Representative fluorescent images showing HLH-30::GFP expression in day 1 young adult worms of indicated genotypes. Worms were raised at non-permissive temperatures (25 °C) forglp-1. Nuclear localization of HLH-30::GFP inglp-1is abolished inglp-1mml-1andglp-1mxl-2animals. (b) Percentage of worms with HLH-30::GFP in the nuclei of intestinal cells at day 1 young adult stage (mean±s.e.m. from 3 biological replicates, >20 worms each, **P<0.01,t-test relative toglp-1). (c) Representative fluorescent images of MML-1::GFP transgenic worms in N2 andglp-1background fed with control L4440::lucRNAi orhlh-30RNAi. Upregulation of nuclear MML-1::GFP inglp-1is abolished onhlh-30knockdown. (d) Nuclear MML-1::GFP intensity relative to N2 fed with control RNAi (mean±s.e.m. from 3 biological replicates, >20 worms each, *P<0.05,t-test relative toglp-1fed with control RNAi). Scale bars, 50 μm. Figure 3: Mutual regulation of MML-1 and HLH-30. ( a ) Representative fluorescent images showing HLH-30::GFP expression in day 1 young adult worms of indicated genotypes. Worms were raised at non-permissive temperatures (25 °C) for glp-1 . Nuclear localization of HLH-30::GFP in glp-1 is abolished in glp-1mml-1 and glp-1mxl-2 animals. ( b ) Percentage of worms with HLH-30::GFP in the nuclei of intestinal cells at day 1 young adult stage (mean±s.e.m. from 3 biological replicates, >20 worms each, ** P <0.01, t -test relative to glp-1 ). ( c ) Representative fluorescent images of MML-1::GFP transgenic worms in N2 and glp-1 background fed with control L4440:: luc RNAi or hlh-30 RNAi. Upregulation of nuclear MML-1::GFP in glp-1 is abolished on hlh-30 knockdown. ( d ) Nuclear MML-1::GFP intensity relative to N2 fed with control RNAi (mean±s.e.m. from 3 biological replicates, >20 worms each, * P <0.05, t -test relative to glp-1 fed with control RNAi). Scale bars, 50 μm. Full size image mml-1/mxl-2 regulates autophagy Autophagy is an essential cellular process critical to multiple longevity pathways, including gonadal longevity [14] , [16] , [17] , [18] , [20] . As HLH-30 regulates autophagy in germline-deficient animals [19] , [28] , [29] , we wondered whether MML-1/MXL-2 also affect autophagy. On autophagy induction, foci containing the LC3 homologues LGG-1 and LGG-2 become more numerous, whereas SQST-1/p62 foci are reduced. We observed that LGG-1::GFP and LGG-2::GFP puncta accumulate in the glp-1 background and this increase depended on mml-1(+) and mxl-2(+) ( Fig. 4a,b and Supplementary Fig. 4a,b ). Furthermore, SQST-1::GFP foci and total protein levels were elevated in glp-1mml-1 and glp-1mxl-2 compared with glp-1 ( Fig. 4c–e ). Previous studies showed that hlh-30 deletion affects autophagic flux and lysosomal function, leading to the accumulation of the lysosomal marker LMP-1::GFP [19] , [28] , [29] . We observed a similar tendency in glp-1mml-1 and glp-1mxl-2 ( Supplementary Fig. 4c ). mml-1 and mxl-2 knockdown did not affect the basal activity of autophagy in wild-type background ( Supplementary Figs. 4d–h ). Altogether, these results suggest that mml-1(+) and mxl-2(+) stimulate autophagy within the gonadal longevity pathway. 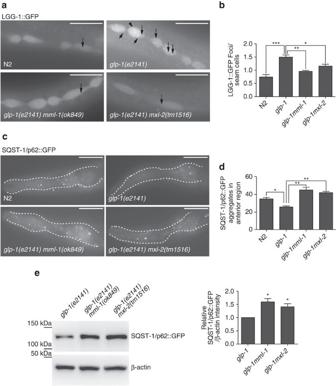Figure 4: MML-1/MXL-2 promote autophagy. (a) Representative fluorescent images of LGG-1::GFP foci in indicated genotypes at L4 stage. LGG-1::GFP puncta are reduced inglp-1mml-1andglp-1mxl-2compared withglp-1. (b) Quantification of LGG-1::GFP puncta in seam cells. The bar represents mean±s.e.m. from 3 biological replicates (>20 worms each).P-value (*P<0.05, **P<0.01) relative to N2 orglp-1was determined byt-test. (c) Representative fluorescent images of SQST-1/p62::GFP transgenic worm of indicated genotypes at L4 stage. SQST-1::GFP aggregates are elevated in double mutants compared withglp-1. (d) Quantification of SQST-1/p62::GFP foci in the pharyngeal region. The bar represents mean±s.e.m. from 3 experiments (>20 worms each).P-value (**P<0.01) relative to N2 orglp-1was determined byt-test. (e) Representative western blotting showing SQST-1::GFP and loading control, b-actin bands in indicated genotypes (left). SQST-1::GFP is elevated inglp-1mml-1andglp-1mxl-2. Quantification of SQST-1::GFP bands is shown (right). Bar graphs show mean±s.e.m. relative toglp-1from three independent experiments. Band intensity of SQST-1::GFP is normalized to loading control, b-actin.P-value (*P<0.05) is determined byt-test relative toglp-1. Scale bars, 20 μm. Figure 4: MML-1/MXL-2 promote autophagy. ( a ) Representative fluorescent images of LGG-1::GFP foci in indicated genotypes at L4 stage. LGG-1::GFP puncta are reduced in glp-1mml-1 and glp-1mxl-2 compared with glp-1 . ( b ) Quantification of LGG-1::GFP puncta in seam cells. The bar represents mean±s.e.m. from 3 biological replicates (>20 worms each). P -value (* P <0.05, ** P <0.01) relative to N2 or glp-1 was determined by t -test. ( c ) Representative fluorescent images of SQST-1/p62::GFP transgenic worm of indicated genotypes at L4 stage. SQST-1::GFP aggregates are elevated in double mutants compared with glp-1 . ( d ) Quantification of SQST-1/p62::GFP foci in the pharyngeal region. The bar represents mean±s.e.m. from 3 experiments (>20 worms each). P -value (** P <0.01) relative to N2 or glp-1 was determined by t -test. ( e ) Representative western blotting showing SQST-1::GFP and loading control, b-actin bands in indicated genotypes (left). SQST-1::GFP is elevated in glp-1mml-1 and glp-1mxl-2 . Quantification of SQST-1::GFP bands is shown (right). Bar graphs show mean±s.e.m. relative to glp-1 from three independent experiments. Band intensity of SQST-1::GFP is normalized to loading control, b-actin. P- value (* P <0.05) is determined by t -test relative to glp-1 . Scale bars, 20 μm. Full size image MML-1/MXL-2 interact with TOR signalling Activated TOR signalling prevents autophagy (by phosphorylation of ATG13) and promotes protein synthesis (through phosphorylation of the p70/S6 kinase and 4EBP) [30] . Recently, it has also been shown to inhibit HLH-30/TFEB nuclear localization and transcriptional activation [19] , [31] , [32] , [33] . Downregulation of TOR signalling provokes opposite effects. A simple hypothesis is that MML-1/MXL-2 regulates autophagy, HLH-30 localization and other activities via TOR signalling. To address this idea, we monitored Thr412/389 phosphorylation of S6Kinase, using anti-phosphopeptide antibodies. Consistent with hyperactivation of TOR, deletion of mml-1 or mxl-2 enhanced phosphorylation of S6K in the glp-1 background ( Fig. 5a ) but not in the wild-type background ( Supplementary Fig. 5a ). Knockdown of let-363 /TOR and TORC1-signalling components lst8/C10H11. 8, daf-15 /raptor and raga-1 restored HLH-30/TFEB nuclear localization in glp-1mml-1 and glp-1mxl-2 backgrounds ( Fig. 5b and Supplementary Fig. 5b ). By contrast, knockdown of the TORC2-specific subunit rict-1/RICTOR had little effect. Collectively, these results indicate that MML-1/MXL-2 represses TOR activity in the gonadal longevity pathway. 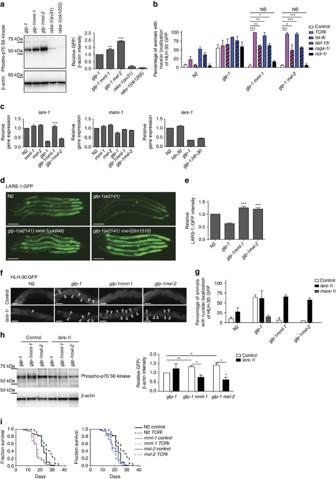Figure 5: MML-1/MXL-2 regulate HLH-30 via regulating TORC1 activity. (a) Western blot analysis of phosphorylation of p70 S6 kinase. Bars show mean±s.e.m. of the band intensity relative toglp-1from three experiments. The band intensity of p70 S6 kinase phosphorylation is normalized to b-actin.P-value (**P<0.01 and ***P<0.001) is determined byt-test relative toglp-1. (b) Bars show the percentage of worms with HLH-30::GFP in the nuclei of intestinal cells at day 1 adult (mean±s.e.m. from 3 biological replicates, >20 worms each). Each RNAi treatment is indicated. Knockdown of TORC1 but not TORC2 components rescues HLH-30 nuclear localization inglp-1mml-1andglp-1mxl-2. Worms of individual genotypes were fed with indicated RNAi from egg onwards and raised at 25 °C.P-values (*P<0.05, **P<0.01 and ***P<0.001) were determined byt-test. (c) qRT–PCR analysis shows thatlars-1but notmars-1is de-repressed inglp-1mml-1. The bar represents mean±s.e.m. from three biological replicates relative to N2.P-value (***P<0.001) was determined by one-way analysis of variance (ANOVA) with Tukey’s test relative toglp-1. (d) Representative fluorescent pictures of LARS-1::GFP. LARS-1::GFP is de-suppressed inglp-1mml-1andglp-1mxl-2. (e) Quantification of LARS-1::GFP in posterior intestinal cells of indicated genotypes. Bars indicate mean±s.e.m. from 3 replicates (>20 worms each).P-value (***P<0.001) is determined byt-test relative toglp-1.(f) Representative fluorescent pictures of HLH-30::GFP in indicated genotypes and RNAi treatments at day 1.lars-1knockdown rescues HLH-30 nuclear localization in double mutants. (g) Percentage of worms with HLH-30::GFP in the nuclei of intestinal cells at day 1 adult (mean±s.e.m. from 3 replicates, >20 worms each). Each RNAi treatment is indicated. (h) A representative western blotting showing phosphorylation of p70 S6 kinase and b-actin (left), and their quantification (right).lars-1knockdown by RNAi significantly reduces the level of phosphorylation of p70 S6 kinase inglp-1mml-1andglp-1mxl-2background. The bar represents mean±s.e.m. from three experiments.P-value (*P<0.05 and **P<0.01) was determined byt-test. (i)mml-1andmxl-2are required for TOR knockdown-mediated longevity. TOR RNAi knockdown was conducted from the day 1 adult stage. Scale bars, 100 μm (d) and 50 μm (f). Figure 5: MML-1/MXL-2 regulate HLH-30 via regulating TORC1 activity. ( a ) Western blot analysis of phosphorylation of p70 S6 kinase. Bars show mean±s.e.m. of the band intensity relative to glp-1 from three experiments. The band intensity of p70 S6 kinase phosphorylation is normalized to b-actin. P -value (** P <0.01 and *** P <0.001) is determined by t -test relative to glp-1 . ( b ) Bars show the percentage of worms with HLH-30::GFP in the nuclei of intestinal cells at day 1 adult (mean±s.e.m. from 3 biological replicates, >20 worms each). Each RNAi treatment is indicated. Knockdown of TORC1 but not TORC2 components rescues HLH-30 nuclear localization in glp-1mml-1 and glp-1mxl-2 . Worms of individual genotypes were fed with indicated RNAi from egg onwards and raised at 25 °C. P -values (* P <0.05, ** P <0.01 and *** P <0.001) were determined by t -test. ( c ) qRT–PCR analysis shows that lars-1 but not mars-1 is de-repressed in glp-1mml-1 . The bar represents mean±s.e.m. from three biological replicates relative to N2. P -value (*** P <0.001) was determined by one-way analysis of variance (ANOVA) with Tukey’s test relative to glp-1 . ( d ) Representative fluorescent pictures of LARS-1::GFP. LARS-1::GFP is de-suppressed in glp-1mml-1 and glp-1mxl-2 . ( e ) Quantification of LARS-1::GFP in posterior intestinal cells of indicated genotypes. Bars indicate mean±s.e.m. from 3 replicates (>20 worms each). P -value (*** P <0.001) is determined by t -test relative to glp-1. ( f ) Representative fluorescent pictures of HLH-30::GFP in indicated genotypes and RNAi treatments at day 1. lars-1 knockdown rescues HLH-30 nuclear localization in double mutants. ( g ) Percentage of worms with HLH-30::GFP in the nuclei of intestinal cells at day 1 adult (mean±s.e.m. from 3 replicates, >20 worms each). Each RNAi treatment is indicated. ( h ) A representative western blotting showing phosphorylation of p70 S6 kinase and b-actin (left), and their quantification (right). lars-1 knockdown by RNAi significantly reduces the level of phosphorylation of p70 S6 kinase in glp-1mml-1 and glp-1mxl-2 background. The bar represents mean±s.e.m. from three experiments. P -value (* P <0.05 and ** P <0.01) was determined by t -test. ( i ) mml-1 and mxl-2 are required for TOR knockdown-mediated longevity. TOR RNAi knockdown was conducted from the day 1 adult stage. Scale bars, 100 μm ( d ) and 50 μm ( f ). Full size image MML-1 regulates TOR signalling through LARS-1 How might MML-1/MXL-2 transcriptionally regulate TOR signalling? From RNA sequencing (RNA-seq) results (below), we found that mml-1 regulates the leucyl-tRNA synthetase lars-1 , whose yeast and mammalian homologues have been recently shown to stimulate TOR via RAG-GTPases [34] , [35] . lars-1 was potently and reproducibly repressed by mml-1(+) in the glp-1 background; accordingly, mutation of mml-1 caused de-repression of the mRNA and increased levels of LARS-1::GFP ( Fig. 5c–e ). Data from the ModEncode project indicate that MML-1 binds directly to the lars-1 promoter ( www.modencode.org ). Similarly, LARS-1::GFP was upregulated in glp-1mxl-2 , (although lars-1 mRNA was not significantly regulated). By contrast, the methionyl-tRNA synthase mars-1 was not obviously regulated in either glp-1mml-1 or glp-1mxl-2 ( Fig. 5c ). Consistent with a role in TOR signalling, we observed that lars-1 RNAi knockdown restored HLH-30/TFEB nuclear localization in the glp-1mml-1 and glp-1mxl-2 backgrounds, whereas knockdown of mars-1 had little effect ( Fig. 5f,g ). In addition, knockdown of lars-1 reduced S6 kinase phosphorylation in glp-1mml-1 and glp-1mxl-2 backgrounds ( Fig. 5h ). Altogether, these observations suggest a model whereby MML-1 downregulates lars-1 and inhibits TOR signalling. Consequently, HLH-30 becomes nuclear localized, initiating transcriptional cascades. Despite the restoration of HLH-30 nuclear localization, knockdown of let-363/ TOR, surprisingly, failed to rescue longevity in the mml-1 and mxl-2 background ( Fig. 5i ). Furthermore, let-363 /TOR knockdown failed to fully restore autophagy or longevity to glp-1mml-1 and glp-1mxl-2 double mutants ( Supplementary Fig. 5c,d ), nor did hlh-30(+) overexpression or raga-1 deletion rescue glp-1mml-1 and/or glp-1mxl-2 short-lived phenotypes ( Supplementary Fig. 5e and Supplementary Table 1 ). These results suggest that MML-1 does not work in a strict linear pathway and may act parallel to or downstream of TOR signalling to mediate additional outputs. By inference, HLH-30 nuclear localization is not sufficient for longevity in this context and MML-1 may promote other key life-extending activities. Shared and preferential targets of MML-1/MXL-2 and HLH-30 To gain further insight into activities of these transcription factors, we compared transcriptomes of wild type, glp-1 , mml-1 , mxl-2 , hlh-30 and double mutants with glp-1 for differentially expressed genes (DEGs) measured by RNA-seq. We used a false discovery rate of 5% when considering DEGs. Hierarchical clustering of gene expression values revealed that biological replicates clustered well together, demonstrating the sample quality ( Supplementary Fig. 6a ). mml-1 or mxl-2 deletion resulted in numerous DEGs that were commonly regulated in either wild type or glp-1 , including both up- and downregulated genes ( Fig. 6a , Supplementary Fig. 6b and Supplementary Table 4 ). For example, 827 genes (382 downregulated and 445 upregulated) were commonly regulated by mml-1 and mxl-2 in the glp-1 background. Each transcription factor also regulated large gene sets independent of the other, in particular mxl-2 deletion, which resulted in hundreds of genes being regulated differently from mml-1 . 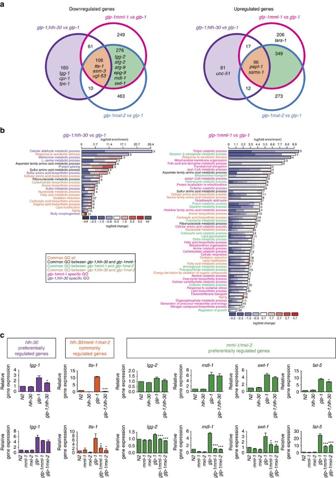Figure 6: Transcriptome analysis reveals preferentially regulated and commonly regulated genes by MML-1/MXL-2 and HLH-30. (a) Venn diagrams depict the numbers of DEGs identified through RNA-seq analysis fromglp-1mml-1versusglp-1,glp-1mxl-2versusglp-1andglp-1;hlh-30versusglp-1. (b) GO enrichment analysis using DAVID. The enrichment (upperxaxis), fold change (colour coding) and number of genes are shown (next to each bar). SeeSupplementary Data 5for details. (c) qRT–PCR analysis confirmshlh-30preferentially regulated genes (lgg-1),hlh-30/mml-1/mxl-2commonly regulated genes (tts-1) andmml-1/mxl-2preferentially regulated genes (lgg-2,mdl-1,swt-1andfat-5). The bar represents mean±s.e.m. from three biological replicates relative to N2.P-value (*P<0.05, **P<0.01 and ***P<0.001) was determined by one-way analysis of variance (ANOVA) with Tukey’s test relative toglp-1. Figure 6: Transcriptome analysis reveals preferentially regulated and commonly regulated genes by MML-1/MXL-2 and HLH-30. ( a ) Venn diagrams depict the numbers of DEGs identified through RNA-seq analysis from glp-1mml-1 versus glp-1 , glp-1mxl-2 versus glp-1 and glp-1;hlh-30 versus glp-1 . ( b ) GO enrichment analysis using DAVID. The enrichment (upper x axis), fold change (colour coding) and number of genes are shown (next to each bar). See Supplementary Data 5 for details. ( c ) qRT–PCR analysis confirms hlh-30 preferentially regulated genes ( lgg-1 ), hlh-30/mml-1/mxl-2 commonly regulated genes ( tts-1 ) and mml-1/mxl-2 preferentially regulated genes ( lgg-2 , mdl-1 , swt-1 and fat-5 ). The bar represents mean±s.e.m. from three biological replicates relative to N2. P -value (* P <0.05, ** P <0.01 and *** P <0.001) was determined by one-way analysis of variance (ANOVA) with Tukey’s test relative to glp-1 . Full size image Gene Ontology (GO) term analysis of glp-1mml-1 versus glp-1 revealed an enrichment of genes implicated in oxidation/reduction, ageing, lipid modification, carbohydrate catabolic process, mitochondrial transport and amine biosynthetic pathway among others ( Fig. 6b and Supplementary Data 1 ). Kyoto Encyclopedia of Genes and Genomes (KEGG) process analysis also revealed enrichment in lysosomal function and fatty acid desaturation ( Supplementary Data 2 ). mxl-2 -dependent DEG in the glp-1 background included similar GO terms as glp-1mml-1 but also included GO terms specific to mxl-2 such as oocyte development, β-oxidation, regulation of translation and cell division among others ( Supplementary Fig. 6c and Supplementary Data 1 ). When we manually interrogated our RNA-seq data, we found several genes regulated by mml-1 and mxl-2 to be involved in autophagy including lgg-2 , atg-2 , atg-9 and epg-9 , and in lysosomal function including ctns-1 , cpr-3 and cpr-5 , many of which we confirmed by quantitative PCR (qPCR) ( Fig. 6c and Supplementary Fig. 6d ). We also found worm homologues of MondoA and ChREBP transcriptional targets involved in glucose and lipid metabolism to be significantly regulated in mml-1 , including the glucose transporter fgt-1 , pyruvate kinase pyk-1 , glycerol 3-phosphate dehydrogenases gpdh-1 , the SREBP homologue sbp-1 and steroyl fatty acid desaturase homologue fat-5 , some of which we confirmed by qPCR ( Fig. 6c and Supplementary Fig. 6d ). A comparison of the MML-1/MXL-2 and HLH-30 transcriptomes in the glp-1 background ( Fig. 6a ) revealed at least three sets of interest: the ‘ hlh-30/mml-1/mxl-2 commonly regulated genes’, ‘ hlh-30 preferentially regulated genes’ and ‘ mml-1/mxl-2 preferentially regulated genes’. (preferentially regulated means that one or the other transcription factor predominately but not exclusively regulates the gene of interest). As predicted, HLH-30 and MML-1/MXL-2 regulated a substantial number of genes in common (106 genes downregulated, 96 genes upregulated, and 28 genes differentially regulated), supporting the idea that they work in overlapping transcriptional cascades. Processes regulated in common to all genotypes included metabolism of xenobiotics, amino acids, fatty acids, amines and nucleosides, as well as oxidation/reduction and ageing ( Fig. 6b ). Commonly regulated genes included tts-1 , sams-1 pept-1 , asm-3 and ugt-53 ( Fig. 6c and Supplementary Fig. 6f ), most of which affect longevity [36] , [37] , [38] ( Supplementary Fig. 6g ). Although both hlh-30 and mml-1/mxl-2 regulated autophagy, they preferentially controlled distinct gene sets: hlh-30 predominately regulated lgg-1/atg-8 and unc-51/atg-1 , whereas mml-1/mxl-2 predominately regulated atg-2 , lgg-2 , atg-9 and epg-9 ( Fig. 6c and Supplementary Fig. 6d,e ). TOR regulates gene expression via a HLH network We next wondered how TOR perturbation would affect the expression of representative genes from the three categories. First, TOR knockdown in the wild type or glp-1 background induced expression of genes such as fat-5 , swt-1 and mdl-1 , which showed preferential dependence on mml-1 and mxl-2 , and less dependence on hlh-30 ( Fig. 7a ). Second, TOR knockdown triggered tts-1 expression in wild type and glp-1 , which was largely dependent on hlh-30 and less dependent on mml-1 / mxl-2 ( Supplementary Fig. 7a ). Third, a handful of mml-1/mxl-2 preferentially regulated autophagy genes such as atg-2 and lgg-2 were rescued by TOR knockdown in an hlh-30 -dependent manner, suggesting that HLH-30 can compensate ( Supplementary Fig. 7a ). Relatedly, double mutation of hlh-30 and mml-1 in many cases (for example, atg-2 and lgg-2 ) abolished TOR-regulated gene expression. Finally, sams-1 , a commonly regulated gene, was largely rescued by TOR knockdown in double- and triple-mutant backgrounds ( Supplementary Fig. 7a ), suggesting that yet other factors can functionally substitute. Taken together, our results suggest that TOR knockdown triggers transcriptional responses through mml-1 , mxl-2 , hlh-30 and other factors, revealing that these HLH transcription factors are major mediators of TOR signalling. 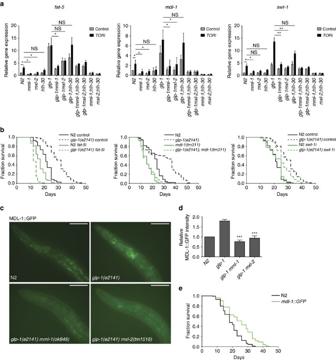Figure 7: MML-1/MXL-2 preferentially regulated genes contribute to gonadal longevity. (a) qRT–PCR analysis of MML-1/MXL-2 preferentially regulated genes after treatment with control or TOR RNAi. The bar represents mean±s.e.m. from three biological replicates relative to N2.P-value (*P<0.05 and **P<0.01) was determined by one-way analysis of variance (ANOVA) with Tukey’s test. (b) Knockdown offat-5,mdl-1andswt-1significantly suppressglp-1longevity. (c) Representative fluorescent images of MDL-1::GFP in indicated strains at day 1 adult. Upregulation of MDL-1::GFP inglp-1background is abolished bymml-1ormxl-2deletion. (d) Quantification of MDL-1::GFP in the head region in indicated genotypes. Bars indicate mean±s.e.m. from 3 biological replicates (>20 worms each).P-value (***P<0.001) was determined byt-test. (e) MDL-1 overexpression extends wild-type lifespan. Scale bars, 50 μm (c). Figure 7: MML-1/MXL-2 preferentially regulated genes contribute to gonadal longevity. ( a ) qRT–PCR analysis of MML-1/MXL-2 preferentially regulated genes after treatment with control or TOR RNAi. The bar represents mean±s.e.m. from three biological replicates relative to N2. P -value (* P <0.05 and ** P <0.01) was determined by one-way analysis of variance (ANOVA) with Tukey’s test. ( b ) Knockdown of fat-5 , mdl-1 and swt-1 significantly suppress glp-1 longevity. ( c ) Representative fluorescent images of MDL-1::GFP in indicated strains at day 1 adult. Upregulation of MDL-1::GFP in glp-1 background is abolished by mml-1 or mxl-2 deletion. ( d ) Quantification of MDL-1::GFP in the head region in indicated genotypes. Bars indicate mean±s.e.m. from 3 biological replicates (>20 worms each). P -value (*** P <0.001) was determined by t -test. ( e ) MDL-1 overexpression extends wild-type lifespan. Scale bars, 50 μm ( c ). Full size image MML-1/MXL-2 regulated genes affect gonadal longevity We reasoned that genes preferentially regulated by mml-1 / mxl-2 should contribute to mml-1 -induced longevity. Focusing on the mml-1 -specific DEGs, we knocked down representative ca . 120 genes that showed upregulation in an mml-1 -dependent manner. A majority of these knockdowns reduced survivorship of glp-1 mutants by up to 30%. Among this set were genes previously implicated in longevity, such as mdl-1 (refs 26 , 39 ), as well novel candidates swt-1 and fat-5. We confirmed that knockdown of these candidates significantly reduced glp-1 longevity in demography experiments ( Fig. 7b and Supplementary Fig. 7b ). Interestingly, we found that MDL-1::GFP was upregulated in germline-deficient animals in a mml-1/mxl-2 -dependent manner ( Fig. 7c,d ). This upregulation contributes to longevity, as mdl-1 overexpression extended wild-type lifespan ( Fig. 7e ) and stimulated expression of specific autophagy genes ( Supplementary Fig. 7c ). Consistent with a role in autophagy, mdl-1 knockdown decreased the number of LGG-1::GFP foci and increased SQST-1/p62::GFP foci in glp-1 background ( Supplementary Fig. 7d–f ). It is interesting to note that mdl-1 knockdown further decreased LGG-1::GFP foci even in glp-1mml-1 and glp-1mxl-2 background, suggesting that mdl-1 additionally regulates autophagy downstream of mml-1/mxl-2 . We also found that mdl-1 overexpression partially rescued the short-lived phenotype of glp-1mml-1 and glp-1mxl-2 ( Supplementary Fig. 7g ). Moreover, the mdl-1 heterodimeric partner mxl-1 was required for glp-1 longevity ( Supplementary Fig. 7h ). These findings support the idea that mml-1/mxl-2 can regulate targets somewhat independently of HLH-30 to affect lifespan and indicate that C. elegans Myc/Mondo family members work in an expansive cascade to regulate gonadal longevity. MondoA and ChREBP regulate TFEB nuclear localization We next asked whether the regulatory cascades observed in C. elegans are conserved in mammals. To test whether MondoA or ChREBP (MondoB) regulate TFEB, we analysed expression and localization in HeLa cells on gene knockdown. First, as observed previously [31] , [32] , amino acid starvation enhanced endogenous TFEB nuclear localization ( Fig. 8a ). When cells were exposed to MondoA small interfering RNA (siRNA), TFEB nuclear localization significantly diminished (control starvation, 79.6±4.1% versus MondoA starvation, 41.6±13.3%; Fig. 8a,b and Supplementary Fig. 8a ). ChREBP siRNA knockdown also modestly affected TFEB nuclear localization (three of four experiments) (control starvation, 71.0±6.2% versus ChREBP starvation, 50.5±7.6%; Fig. 8a,c and Supplementary Fig. 8b ). Correlatively, TFEB direct target genes showed reduced expression, although surprisingly, with some specificity: MondoA knockdown more dramatically affected ctsb , whereas ChREBP knockdown blunted the expression of vps11 ( Fig. 8d and Supplementary Fig. 8c ). Finally, TFEB knockdown led to decreased steady state levels of MondoA and ChREBP in cell culture ( Fig. 8e ). These findings indicate that mammalian MondoA/ChREBP and TFEB mutually regulate one another. 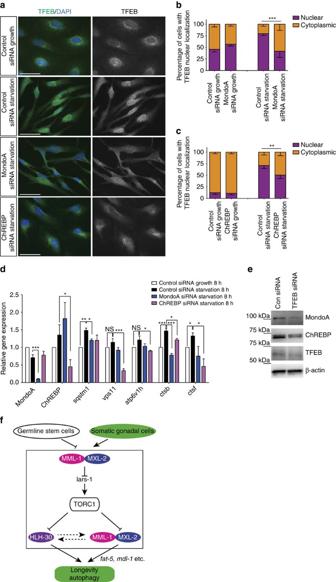Figure 8: MondoA and ChREBP knockdown compromise TFEB nuclear localization and target gene expression. (a) Representative fluorescent images of TFEB nuclear localization on control, MondoA or ChREBP knockdown in HeLa cells. Starvation-induced TFEB nuclear localization (4 h) is impaired by MondoA and ChREBP siRNA knockdown. (b) Quantification of TFEB nuclear localization on control or MondoA knockdown. (c) Quantification of TFEB nuclear localization on control or ChREBP knockdown. Bars indicate mean±s.e.m. from four biological replicates.χ2-test, **P<0.01 ***P<0.001 (b,c) (d) TFEB target gene expression is affected on MondoA and ChREBP knockdown. The bar represents mean±s.e.m. from five experiments relative to control siRNA 8-h growth condition.P-value (*P<0.05 and ***P<0.001) was determined by one-way analysis of variance (ANOVA) with Tukey’s test relative to control siRNA growth or starvation condition. (e) Representative western blotting showing that TFEB knockdown leads to decreased steady-state levels of MondoA and ChREBP. (f) A working model based on the current study. MML-1 is upregulated on germline removal. Activated MML-1/MXL-2 represses TOR activity by downregulatinglars-1, leading to the nuclear localization of HLH-30. MML-1/MXL-2 also work downstream of TOR and activate preferential targets such as MDL-1, to regulate autophagy and longevity. HLH-30 also upregulates MML-1 through an unknown mechanism (see also Discussion). Scale bars, 50 μm (a). Figure 8: MondoA and ChREBP knockdown compromise TFEB nuclear localization and target gene expression. ( a ) Representative fluorescent images of TFEB nuclear localization on control, MondoA or ChREBP knockdown in HeLa cells. Starvation-induced TFEB nuclear localization (4 h) is impaired by MondoA and ChREBP siRNA knockdown. ( b ) Quantification of TFEB nuclear localization on control or MondoA knockdown. ( c ) Quantification of TFEB nuclear localization on control or ChREBP knockdown. Bars indicate mean±s.e.m. from four biological replicates. χ 2 -test, ** P <0.01 *** P <0.001 ( b , c ) ( d ) TFEB target gene expression is affected on MondoA and ChREBP knockdown. The bar represents mean±s.e.m. from five experiments relative to control siRNA 8-h growth condition. P -value (* P <0.05 and *** P <0.001) was determined by one-way analysis of variance (ANOVA) with Tukey’s test relative to control siRNA growth or starvation condition. ( e ) Representative western blotting showing that TFEB knockdown leads to decreased steady-state levels of MondoA and ChREBP. ( f ) A working model based on the current study. MML-1 is upregulated on germline removal. Activated MML-1/MXL-2 represses TOR activity by downregulating lars-1 , leading to the nuclear localization of HLH-30. MML-1/MXL-2 also work downstream of TOR and activate preferential targets such as MDL-1, to regulate autophagy and longevity. HLH-30 also upregulates MML-1 through an unknown mechanism (see also Discussion). Scale bars, 50 μm ( a ). Full size image Numerous transcriptional factors mediate the outputs of the major longevity pathways [1] ; yet, how they form coherent transcriptional regulatory networks is not understood. The gonadal longevity pathway is a rich multi-layered regulatory network, reflecting the intense evolutionary pressure to propagate an intact germline in the face of changing environments, nutrient conditions and physiologic milieus. In this work, we unravel a core regulatory node governing C. elegans gonadal longevity. We have found that the HLH Mondo/Max-like complex MML-1/MXL2 is required to promote longevity of germline-less animals. This complex also promotes longevity triggered by reduced TOR and insulin/IGF signalling, reduced mitochondrial respiration in some measure, as well as reportedly by dietary restriction [26] . Thus, MML-1/MXL-2 is among a handful of select factors working at the convergence of major longevity pathways. Most interestingly, we have discovered that the MML-1/MXL-2 complex dramatically stimulates nuclear localization and activity of the TFEB homologue HLH-30, a convergent regulator of autophagy, lysosome biogenesis, fat metabolism and longevity [19] , [28] , [29] , via TOR signalling. In germline-less animals, MML-1/MXL-2 transcriptionally repress the leucyl-tRNA synthase LARS-1, a positive effector of the TOR signalling pathway [34] , [35] , which results in HLH-30 nuclear localization and activity (see Model; Fig. 8f ). HLH-30 itself promotes upregulation of MML-1 in the germline-less glp-1 background. Our findings expand the functional outputs of MML-1/MXL-2 complex as key regulators of autophagy, TOR and TFEB signalling. Importantly, we found that aspects of these regulatory relationships are evolutionarily conserved: mammalian homologues MondoA and ChREBP stimulate TFEB nuclear localization on amino acid starvation in cell culture. Thus, MML-1/Mondo and HLH-30/TFEB form a tight regulatory ensemble linked through TOR signalling, as well as presumably through E-box elements commonly bound by HLH transcription factors. bHLH transcription factors regulate proliferation, growth, development and metabolism, and form an extensive interlocking network through heterodimerization and similar DNA-binding sites. The C. elegans HLH transcription factors have been assembled into an incipient network and Myc/Mondo complexes bind to similar E-box elements (CACGTG) as HLH-30/TFEB [22] , [23] , [40] . Consistent with interlinked regulatory cascades, our transcriptome data indicate that MML-1, MXL-2 and HLH-30 substantially overlap in target gene expression, but also have preferential outputs. MML-1 and MXL-2 are well known to work in a complex [23] , [40] and accordingly show considerable overlap in their transcriptomes, tissue distribution and their mutant phenotypes. Surprisingly, more genes were upregulated than downregulated in the mutants, suggesting that this ‘activation complex’ may well have potent repressive activity. MXL-2 shows broader transcriptomic changes than MML-1, indicating participation in other complexes. Supporting the idea of independence, mml-1 and mxl-2 mutants exhibit somewhat different patterns of genetic epistasis, for example, mml-1 is required for isp-1 longevity, whereas mxl-2 is not. Perhaps this difference reflects our observed association of MML-1 with the mitochondria and the enrichment of mitochondria GO terms from mml-1 transcriptome analysis. MML-1 and HLH-30 also show significant transcriptional overlap but preferentially regulate distinct gene sets. Overlapping-regulated processes include amino acid, fat, amine, nucleoside and xenobiotic metabolism, oxidation/reduction and others, possibly pinpointing processes important for longevity ( Fig. 6 ). Interestingly, sulfur amino acid metabolism has been linked to methionine restriction and H 2 S metabolism, which affect life span [41] . Another common striking output is tts-1 , a long non-coding RNA that represses protein synthesis and affects multiple longevity pathways [36] , [37] , [38] . As mml-1 and hlh-30 represent convergent regulators of longevity, further functional dissection of their transcriptomes should illuminate core processes for lifespan extension. ModEncode data indicate that MML-1 and HLH-30 often reside at the same promoters [23] , [40] , [42] . Currently, it is not known whether the two factors bind independently or cooperatively, act in series as part of transcriptional cascades or work together in a complex. In addition, their temporal dynamics and whether they function in a tissue- or stage-specific manner remain to be elucidated. Future work to identify transcriptional complexes and their binding sites in the genome (chromatin immunoprecipitation sequencing) in the context of ageing should clarify these issues. Although HLH-30 overexpression modestly extends lifespan [19] , our data indicate that HLH-30 activity is not sufficient to promote longevity in the gonadal pathway. Although knockdown of TOR signalling partially bypassed the mml-1/mxl-2 requirement for HLH-30 nuclear localization and activity in the glp-1 background, it was, surprisingly, unable to drive autophagy and longevity. This observation indicates that these factors act within partially overlapping networks, rather than a strict linear pathway, and that mml-1/mxl-2 leverages key processes for longevity. Accordingly, mml-1 preferential transcriptional targets fat-5 , swt-1 and mdl-1 also facilitated longevity. Previously, Goudeau et al . [13] showed that fat-5 deletion does not affect glp-1 longevity, which is contradictory to our results ( Fig. 7b and supplementary Fig. 7b ). Although the exact cause for this difference is unknown, Goudeau et al . [13] used bacterial strain HT115, whereas we used OP50, suggesting that the food source may be responsible. mml-1 and hlh-30 also regulated the process of autophagy in common but preferentially affected distinct components: mml-1 mainly affected atg-2 and lgg-2 , whereas hlh-30 affected atg-1 and lgg-1. Conceivably, other mml-1/mxl-2 -enriched processes such as glycerol or mitochondrial metabolism also contribute. Our data suggest that MML-1 represents an ancestral MondoA/ChREBP transcription factor conserved at many levels, which can inform mammalian metabolism and ageing. First, MML-1 and Mondo share common protein-domain structure including nuclear localization and glucose regulatory domains at the amino terminus and the bHLH-Zip domains at the carboxy terminus [23] . Second, mml-1 target genes are remarkably similar to those regulated by mammalian counterparts including genes involved in sugar transport ( fgt-1 ), fatty acid desaturation ( fat-5 ), pyruvate kinase ( pyk-1 ), sterol regulatory binding protein ( sbp-1 ) and glycerol-3-phosphate dehydrogenase ( gpdh-1 ) [24] , [27] , [43] . Whether C. elegans MML-1 senses glucose metabolites and has an impact on glycolysis and lipogenesis remain to be tested. Conversely, novel genes and processes regulated by C. elegans MML-1/MXL-2 (for example, autophagy, lysosomal and mitochondrial function) are plausible targets to further test in the mammalian system. Third, our work here reveals an evolutionarily conserved interrelationship between MONDO and TFEB. In response to germline removal, MML-1/MXL-2 promotes HLH-30 nuclear localization and activation; conversely, HLH-30 also upregulates MML-1 in germline-less animals. Similarly, MondoA and ChREBP facilitate TFEB nuclear localization and gene expression in response to amino acid starvation in cell culture, and TFEB knockdown reduced MondoA and ChREBP expression, revealing that the homologous transcription factors show mutual regulation. MondoA and ChREBP furthermore regulated TFEB gene targets, revealing a novel role in lysosomal function but, unexpectedly, affected distinct genes, perhaps reflecting their functional or temporal diversification. Other transcription factors working within the gonadal pathway show dependence: DAF-12/steroid receptor signalling facilitates DAF-16/FOXO nuclear localization [44] , [45] and MXL-2 stabilizes MML-1 (ref. 23 ). Speculatively, such positive reinforcement could stabilize a fragile interdependent network architecture to maintain coherent states geared towards reproduction or survival. Fourth, MML-1/MXL-2 and MondoA/ChREBP function are intimately linked to TOR signalling. On the one hand, our data suggest that MML-1 suppresses TOR in germline-less animals; mml-1 loss-of-function hyperactivates TOR through upregulation of lars-1 and perhaps other factors, resulting in increased S6K activity, decreased autophagy and impaired nuclear localization of HLH-30. On the other hand, mml-1 loss often suppressed transcriptional changes and longevity arising from TOR knockdown. Thus, MML-1 may act both upstream, to transcriptionally repress TOR signalling, and downstream, to mediate the output of reduced TOR signalling. By inference, MML-1 may work in a feedback loop to limit TOR signalling. Transcription factors genetically regulated by C. elegans TOR are limited to DAF-16/FOXO, SKN-1/NFE2, PHA-4/FOXA and HLH-30/TFEB [19] , [46] , [47] , but mechanistic links still remain obscure. Thus, the identification of MML-1/MXL-2 as potent suppressors of TOR-induced autophagy, longevity and gene expression reveals these transcription factors as critical outputs of this nutrient-sensing pathway. Although MondoA and ChREBP are best known as glucose sensors that signal replete states, our studies suggest a potential role under nutrient limitation. Accordingly, Ayer and colleagues [48] have recently shown that mammalian MondoA suppresses mammalian TOR (mTOR) through upregulation of the TXNIP (thioredoxin-interacting protein), a regulator of glucose uptake and cellular redox signalling. Conversely, mTOR binds and sequesters MondoA activity in response to reactive oxygen species (ROS) and mTOR knockdown stimulates specific MondoA gene targets. MondoB/ChREBP also binds to mTOR. Whether MML-1/MondoA/ChREBP are direct targets of TOR phosphorylation is currently unknown. It is also unclear how germline removal triggers MML-1 activation: is it through glucose or related metabolites, TOR, ROS signalling or other signals? In this regard, it is intriguing that both MML-1 and MondoA are not only nuclear localized but are also present in the mitochondria, a site of ROS production [27] . Preliminary data also suggest that a fraction of MML-1 resides at the lysosome (S.N. and A.A., unpublished observation), a critical site of TOR action and TFEB localization [31] , [33] . Finally, our studies highlight a convergent core role for Myc/Mondo complexes in the regulation of animal longevity. Previous work implicated mml-1/mxl-2 in IIS and dietary restriction pathways [26] ; our studies greatly expand this role to longevity induced by HLH-30, germline loss, decreased TOR signalling and, in part, mitochondrial longevity. In recent times, Sedivy and colleagues [49] showed that Myc +/− heterozygote mice exhibit healthier lipid metabolism, increased physical activity, higher metabolic rate, less age-related pathologies and enhanced longevity. Molecular correlates include reduced IGF, increased AMPK, decreased AKT, mTOR and S6K activity, and protein synthesis. Evidently, various members of the Myc/Mondo HLH transcription factor family function to regulate metazoan lifespan through major growth factor and energy- and nutrient-sensing pathways. It is striking that among target genes regulated by MML-1/MXL-2 is yet another member of the Myc subfamily, MDL-1, encoding the Mad-like homologue, which we found to be required for germline-less longevity, and whose overexpression is sufficient to extend life. We therefore suggest that Myc/Mondo HLH transcription factors comprise an extensive cascade regulating metabolism and longevity. Disentangling their distributed and shared responsibilities, as well as cross-regulation, and understanding how these interactions specifically impact metabolism and ageing will be fascinating to explore. C. elegans growth conditions Nematodes were cultured using standard techniques at 20 °C on nematode growth medium agar plates with the Escherichia coli strain OP50, unless otherwise noted. Strains with glp-1(e2141) background were maintained at 15 coli °C and grown at 25 °C to induce germline-deficient phenotype. All strains used in this study are listed in Supplementary Table 2 . Lifespan assays Synchronized eggs were obtained by 4–6 coli h egg lay. When they reached day 1 adults, lifespan experiments were set up at a density of 15–20 animals per plate and carried out at 20 °C. These animals were transferred to new plates every other day. Survivorships of worms were also counted every other day. Death was scored as the absence of any movement after stimulation by a platinum wire. For lifespan experiments using isp-1(qm150) strains, egg lays were conducted 3 days before that of other strains, to obtain day 1 adults at the same time. Worms undergoing internal hatching, bursting vulva or crawling off the plates were censored. For all experiments, strains and/or conditions were blinded. For the ablation of germline precursor cells, newly hatched L1 worms were anaesthetized in 0.5% phenoxypropanol in M9 buffer. Z2/Z3 germline precursor cells were ablated by laser microsurgery (Micropoint) and successful ablations were confirmed under the dissecting microscope at day1 adult stage. The controls (mock ablated) were also anaesthetized in parallel with experimental animals and included for lifespan assay. For lifespan experiments using the glp-1 strain, all strains were raised at 25 °C for 2 days, to induce the glp-1 phenotype after the egg lay at 15 °C. Subsequently, lifespan experiments were resumed at 20 °C. In some cases, we observed a relatively long median lifespan of N2 under these conditions, presumably due to hormesis effects of the temperature shift. For all lifespan experiments, strains and/or conditions were blinded. Statistical analyses were performed with the Mantel–Cox log rank method in Excel (Microsoft). RNA interference RNAi was conducted by feeding HT115 (DE3) bacteria transformed with L4440 vector that produces double-stranded RNA against the targeted gene. Synchronized eggs obtained by egg lay were put on corresponding RNAi plates containing isopropyl-β- D -thiogalactoside and ampicillin. RNAi clones were available from the Ahringer or Vidal RNAi library. let-363/TOR RNAi clone was a gift from Dr Hansen (Sanford-Burnham Medical Research Institute). Empty vector (L4440) or Luciferase (L4440::Luc) RNAi were used as non-targeting control. glp-1(e2141) suppressor screening was conducted using transcription factor RNAi library [7] . glp-1(e2141) worms were synchronized by tight egg lay and treated by control RNAi and RNAi targeting transcription factors. The survivorship at day 25 was used as an estimate of longevity. RNAi suppressor screening was replicated twice and only the candidates that show reproducible results were taken into consideration for further analysis. For all genes that are targeted by RNAi in this study, we indicated ‘i’ after the gene name. Plasmid construction and transgenesis mml-1 :: GFP translational fusion construct that contains 4-kb promoter and mml-1 coding sequence is a kind gift from Dr. Ayer [23] . For mxl-2 :: GFP and lars-1 :: GFP translational fusion constructs, mxl-2 and lars-1 4-kb endogenous promoter plus coding sequence were cloned into pDC4 vector, which contain an enhanced green fluorescent protein (GFP) tag, respectively. Microinjection of these constructs was carried with the co-injection marker myo-2p :: mCherry to generate dhEx966 ( mml-1p::mml-1::GFP , myo-2p::mCherry ), dhEx967 ( mml-1p::mml-1::GFP , myo-2p::mCherry ), dhEx1037 ( mxl-2p::mxl-2::GFP , myo-2p::mCherry ) and dhEx1031 ( lars-1p::lars-1::GFP , myo-2p::mCherry ). We obtained mdl-1 ::GFP from the CGC and outcrossed the strain with our wild type, to use for lifespan and microscopy experiments. mdl-1 ::GFP strain, unc-119(ed3) III; wgIs106[mdl-1::TY1::EGFP::3xFLAG+unc-119(+)] , which contains the endogenous mdl-1 promoter and coding region, was originally made by TransgeneOme project ( https://transgeneome.mpi-cbg.de/transgeneomics/index.html ). RNA extraction and qRT–PCR Worms and cell samples were harvested in TRIzol (Invitrogen). Total RNA was extracted using RNeasy or miRNAeasy kit (QIAGEN). Complementary DNA was generated using iScript (Bio-Rad). Quantitative reverse transcriptase–PCR (qRT–PCR) was performed with Power SYBER Green (Applied Biosystems) on a ViiA 7 Real-Time PCR System (Applied Biosystems). Four technical replicates were performed in each reaction. ama-1 and/or cdc-42 (for worms), and GAPDH (for cells) were used as an internal control. Primer sequences are listed in Supplementary Table 3 . Western blotting Worms at L4 or day 1 adult were lysed in worm lysis buffer (50 mM Tris-HCl pH 7.4, 150 mM NaCl, 1 mM EDTA, 0.1% NP-40, protease and phosphatase inhibitor cocktail (Roche)) using a dounce homogenizer. [50] After the centrifugation, the supernatants were used for protein measurement and subsequent western blotting analysis. Worm protein lysates were separated by SDS–PAGE (Bio-Rad) and transferred to polyvinylidene difluoride membrane (Bio-Rad). Membranes were incubated with specific primary antibodies. Primary antibodies and dilutions used for worm western blotting are as follows: mouse anti-GFP (1/2,500, Clontech, 632380), rabbit anti-phospho-p70 S6 kinase (Thr412) (1/500, Millipore, 07-018), which detects conserved residue Thr404 in worms, and mouse anti-b-actin (1/10,000, Abcam, ab8224). The band intensity was quantified by Image J (version 1.48) ( http://imagej.nih.gov/ij/ ). The uncropped western blotting results are shown in Supplementary Fig. 9 . Microscopy and quantification of GFP To monitor the autophagy activity, LGG-1::GFP, SQST-1/p62::GFP and LGG-2::GFP animals were anaesthetized in 0.1% sodium azide and GFP puncta in the seam cells (LGG-1::GFP), in the pharyngeal region (SQST-1/p62::GFP) or in the tail region (LGG-2::GFP) were counted at L4 stage after taking pictures using a Zeiss Axio Imager Z1 microscope. For quantification of MML-1::GFP, MXL-2::GFP, HLH-30::GFP, DAF-16::GFP and MDL-1::GFP, animals were anaesthetized in 1 mM Levamisole or 0.1% sodium azide and pictures were taken at day 1 adult stage at the same exposure time using a Zeiss Axio Imager Z1 microscope. GFP intensity in the intestine (MML-1::GFP, MXL-2::GFP, HLH-30::GFP and DAF-16::GFP) or the head region (MDL-1::GFP) was measured and quantified using Image J (version 1.48). For LARS-1::GFP quantification, animals were aligned on pre-cooled unseeded plates and pictures were taken at day 1 adult stage using Leica M165 FC microscopy. LARS-1::GFP intensity of posterior intestine was measured and quantified using image J (version 1.48). For the nuclear localization assay of HLH-30::GFP and MML-1::GFP, animals were anaesthetized in 0.1% sodium azide at day 1 adult stage and the numbers of animals carrying nuclear HLH-30::GFP or MML-1::GFP were quantified. For all microscopy experiments, more than 20 worms were scored in each experiment and all experiments were repeated at least three times. Mitochondrial staining Synchronized eggs were incubated on nematode growth medium plates containing 500 nM MitoTracker Deep Red (Molecular Probe) for 2 days. The worms were washed by M9 and mounted on agarose pads. Pictures were taken by Leica confocal microscopy SP5 X. The deconvolution was conducted using Huygens Professional (Scientific Volume Imaging), to examine localization of MML-1::GFP and MXL-2::GFP to mitochondria. RNA sequencing For each genotype, more than 300 day 1 adult worms were collected in Trizol in three independent biological replicates. One microgram of of RNA was extracted using miRNAeasy Mini Kit (QIAGEN). polyA+ mRNA was isolated from 500 ng total RNA with NEBNext Poly(A) mRNA Magnetics Isolation Module (New England Biolabs). RNA-seq libraries were prepared with the NEBNext Ultra Directional RNA Library Prep Kit for Illumina (New England Biolabs). Quality and quantity was assessed at all steps by capillary electrophoresis (Agilent Bioanalyser and Agilent Tapestation). Libraries were quantified by fluorometry, immobilized and processed onto a flow cell with a cBot (Illumina) followed by sequencing-by-synthesis with TruSeq v3 chemistry on a HiSeq2500 at the Max Planck Genome Center (Cologne, Germany). Reads were trimmed for adapter and barcodes using the Flexbar version 2.5 software [51] . Alignment of the reads was done using the Tophat version 2.0.13 software against the Wormbase genome (WBcel235_79). The Tuxedo/cufflinks version 2.2.1 software pipeline was used to perform differential gene expression analysis on pairwise comparisons of the different samples. Dispersion was calculated per condition (genotypes) and differential expressed genes ( q -value<0.05) of each pairwise comparison were identified. GO annotation and enrichment analysis was performed using the DAVID bioinformatics resources database. Cell culture experiments HeLa (P5-P10) cells (American Type Culture Collection, USA; ATCC-CCL-2) were maintained in DMEM medium (Gibco), supplemented with 10% fetal bovine serum (Gibco). Transfections of MondoA (Santa Cruz Biotechnology), ChREBP (Santa Cruz Biotechnology) and TFEB (GE Dharmacon) siRNA with respective control siRNAs were performed using INTERFERin (Polyplus Transfection) according to the manufacturer’s instruction. For TFEB nuclear localization assay, cells were starved in the starvation medium (140 mM NaCl, 1 mM CaCl 2 , 1 mM MgCl 2 , 5 mM glucose, 1% BSA and 20 mM HEPES, pH 7.4) [52] for 4 h (for immunohistochemistry and western blotting) and fixed by 4% paraformaldehyde followed by MeOH fixation. Immunohistochemistry was performed using anti-TFEB antibody (1/500, rabbit or goat, Cell Signaling, #4240 or Abcam ab2636, respectively) followed by anti-rabbit or anti-goat secondary Alexa 488 antibody (1/500, donkey, ThermoFisher Scientific, A-11055) incubation. For each experimental condition, more than 100 cells were scored for their TFEB nuclear localization in a blinded manner and in at least 3 different biological replicates. For each biological replicate, the quantity of MondoA or ChREBP gene knockdown was measured by western blottings. For western blotting, cells were collected in RIPA buffer (Cell Signaling) with cOmplete protease inhibitor (Roche). The following antibodies and concentrations were used: anti-MondoA (1/1,000, rabbit, Santa Cruz Biotechnology, sc-133397), anti-ChREBP (1/1,000, goat, Santa Cruz Biotechnology, sc-21189), anti-TFEB (1/1,000, rabbit, Novus, NB100-1030) and anti-b-actin (1/10,000, mouse, Cell Signaling, #3700). For qRT–PCR experiments, cells were starved for 8 h in starvation medium and collected in Trizol (Roche). qPCR primers used for gene expression analyses are listed in Supplementary Table 3 . Statistical analysis Results are presented as mean±s.e.m. Statistical tests were preformed with either one-way analysis of variance with Tukey’s test or t -test using GraphPad Prism (GraphPad Software) or Excel (Microsoft Office 2011). Accession codes: RNA-seq data have been deposited in the ArrayExpress database under accession code E-MTAB-3686 . How to cite this article: Nakamura, S. et al . Mondo complexes regulate TFEB via TOR inhibition to promote longevity in response to gonadal signals. Nat. Commun. 7:10944 doi: 10.1038/ncomms10944 (2016).